Long-term carbon loss in fragmented Neotropical forests Tropical forests play an important role in the global carbon cycle, as they store a large amount of carbon (C). Tropical forest deforestation has been identified as a major source of CO 2 emissions, though biomass loss due to fragmentation—the creation of additional forest edges—has been largely overlooked as an additional CO 2 source. Here, through the combination of remote sensing and knowledge on ecological processes, we present long-term carbon loss estimates due to fragmentation of Neotropical forests: within 10 years the Brazilian Atlantic Forest has lost 69 (±14) Tg C, and the Amazon 599 (±120) Tg C due to fragmentation alone. For all tropical forests, we estimate emissions up to 0.2 Pg C y −1 or 9 to 24% of the annual global C loss due to deforestation. In conclusion, tropical forest fragmentation increases carbon loss and should be accounted for when attempting to understand the role of vegetation in the global carbon balance. Vegetation plays an important role within the global carbon cycle, storing approximately 610 Pg carbon (C) above ground, that is, almost the same amount as that stored in the atmosphere (750 Pg C) (refs 1 , 2 , 3 , 4 , 5 ). Most of the carbon bound in vegetation is tied to tropical forests [1] , [2] , [3] , [4] , [6] . However, there are large uncertainties in the quantification of the carbon balance of tropical forests [7] , [8] , [9] , [10] , [11] , [12] , [13] , [14] , [15] , due to processes that do not destroy the forest but alter forest structure, which have not been well quantified [8] , [9] , [10] , [16] , [17] , [18] . Processes leading to forest degradation [8] , [11] , [19] , [20] include fragmentation, selective logging and conversion of pristine into secondary forests [16] , [19] , [21] , [22] . One of these processes, which are mostly unconsidered for the carbon balance of the vegetation in the global carbon cycle, is the change in carbon emissions following fragmentation of tropical forests—which results in the creation of additional forest-edge areas. Such carbon emissions are often unconsidered, because they are difficult to quantify, especially at larger spatial (for example, at biome-wide or continental) and temporal (for example, decades) scales. Nevertheless, as habitat loss may increase in tropical regions, in addition to the biodiversity decline [23] and the impact on several key ecological processes [24] , the relevance of fragmentation processes may increase in the future. In the tropics, forest fragmentation increases tree mortality within the first 100 m of the forest edge [21] , [22] , [25] , [26] , [27] , [28] , [29] , [30] , causing additional long-term carbon loss. Carbon losses depend not only on the area of the forest patches, but also on the shape. Field studies, such as estimates of local above-ground tree biomass and tree mortality due to fragmentation [25] , [26] , [29] , [30] , [31] , generally have time horizons too short for the direct monitoring of long-term carbon loss in forest fragments [27] , [29] , [30] , [31] , but provide important input for modelling temporal effects. Modelling studies showed that increased mortality at edges of forest fragments is by far the most influential factor driving the dynamics of trees, especially in smaller forest fragments <25 ha (ref. 32 ). To advance our understanding of carbon loss due to forest fragmentation at larger spatial scales, we combine remote-sensing data with estimations of carbon losses in tropical forest fragments obtained via a process-based forest model. We are aware of the complexity of this challenge (heterogeneous forest biomass distribution, dynamic land use, heterogeneous forest fragments and unknown parameters of forest dynamics for different locations). Thus, our study presents a first step towards a possible strategy of how this challenge may be tackled in principle. This approach can be generalized and can be complemented in the future, when more empirical information became available. The main aims of this paper are twofold: first, to estimate the biome-wide (Brazilian Atlantic Forest and the Amazon Forest) amount of carbon losses as consequence of increased tree mortality in forest fragments in a generalizable manner; and second, to show exemplarily, how empirically known spatial processes such as increased tree mortality at fragment edges can be integrated into large-scale remote-sensing analyses. In conclusion, we provide a generalizable strategy enabling the use of the knowledge of local ecological processes for large-scale analysis, and we show that tropical forest fragmentation increases carbon loss. Thus, the consideration of fragmentation processes will provide a better understanding of the role of vegetation in the global carbon balance. Biome-wide spatial distribution of forest fragments The spatial distribution of forests and forest fragments show opposing trends in the two biomes ( Figs 1 and 2 ). The Brazilian Atlantic Forest ( Fig. 1 , and Supplementary Fig. 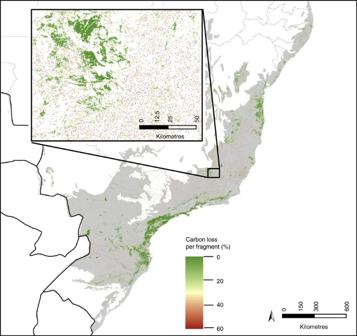Figure 1: Spatial forest fragment distribution for the Brazilian Atlantic Forest. Spatial distribution of the Brazilian Atlantic Forest fragments (data from 2005) and their estimated carbon loss due to fragmentation. Colour ranges indicate the estimated relative carbon loss due to fragmentation (over a period of 30 years, see alsoSupplementary Fig. 1). Black lines indicate national borders, pink lines indicate Brazilian state limits and grey shading indicates the study area. 1 , based on Landsat data with 50 m resolution) is strongly deforested, with the remaining forests—covering approximately 11% of its original cover—distributed heterogeneously across 245,173 mainly small fragments with a mean fragment size of 64 ha ( Table 1 ) and a few extended areas of continuous forest. The Amazon Forest ( Fig. 2 )—with a remaining forest cover of 68% based on the MODIS analysis with a target resolution of around 250 m (see Methods)—results in 77,038 fragments with a mean fragment size of 8,376 ha for the whole Amazon ( Table 1 ). Overall, the Amazon still retains large blocks of little disturbed forests, with forest fragments being concentrated in the southern and eastern part of Amazonia. The size distribution of fragments up to 10 4 ha does not differ qualitatively ( Fig. 3 ), nevertheless the spatial distributions of forest fragments of the Amazon Forest and the Brazilian Atlantic Forest are completely opposite: the Atlantic Forest is deforested with a lot of remaining small fragments, whereas the Amazon consists of contiguous forests with spots of deforestation in between, except for the arc of deforestation in the southern and the eastern part of the Amazon. Figure 1: Spatial forest fragment distribution for the Brazilian Atlantic Forest. Spatial distribution of the Brazilian Atlantic Forest fragments (data from 2005) and their estimated carbon loss due to fragmentation. Colour ranges indicate the estimated relative carbon loss due to fragmentation (over a period of 30 years, see also Supplementary Fig. 1 ). Black lines indicate national borders, pink lines indicate Brazilian state limits and grey shading indicates the study area. 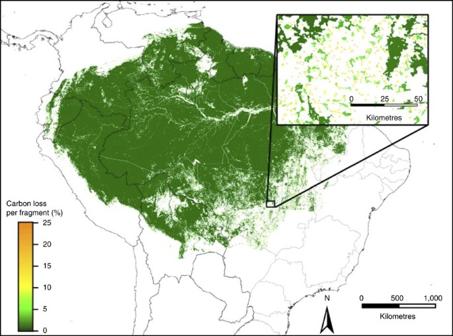Figure 2: Spatial forest fragment distribution for the Amazon Forest. Spatial distribution of tropical forest fragments in the Amazon Forest (data from 2009) and their estimated carbon loss due to fragmentation. Colour ranges indicate the estimated relative carbon loss due to fragmentation (over a period of 30 years). National borders and Brazilian state limits are indicated by black and light grey lines respectively. Full size image Figure 2: Spatial forest fragment distribution for the Amazon Forest. Spatial distribution of tropical forest fragments in the Amazon Forest (data from 2009) and their estimated carbon loss due to fragmentation. Colour ranges indicate the estimated relative carbon loss due to fragmentation (over a period of 30 years). National borders and Brazilian state limits are indicated by black and light grey lines respectively. Full size image Table 1 Overview on remote-sensing results and estimated carbon losses. 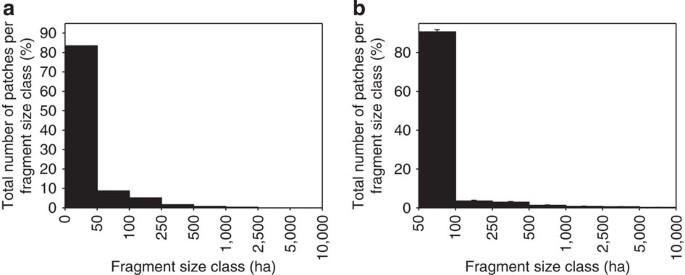Figure 3: Forest fragment frequency distribution for the Atlantic and the Amazon Forest. Data are shown for (a) the Brazilian Atlantic Forest and for (b) the Brazilian or Legal Amazon Forest, respectively (bar, mean; error bars, range out of both analysis of the PRODES dataset). Full size table Figure 3: Forest fragment frequency distribution for the Atlantic and the Amazon Forest. Data are shown for ( a ) the Brazilian Atlantic Forest and for ( b ) the Brazilian or Legal Amazon Forest, respectively (bar, mean; error bars, range out of both analysis of the PRODES dataset). Full size image Simulation results Simulated forest dynamics after fragmentation of an old-growth forest indicate that structural changes within the forest lead to a new equilibrium of above-ground forest carbon after approximately 100 years ( Supplementary Fig. 2 ). Most of the changes and carbon loss occurred within the first 30 years. Carbon loss relative to undisturbed forests is highest for fragments smaller than 10 ha ( Fig. 4 and Supplementary Fig. 2 , with up to approximately 50% carbon loss within a 30-year period after fragmentation). 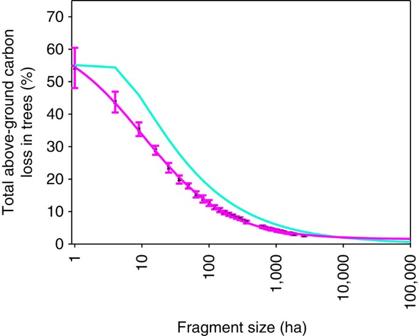Figure 4: Model comparison for the estimated long-term impact of fragmentation on forests. Relative carbon loss per fragment over 30 years for different fragment sizes. Shown are results of a simple edge-effect model (turquoise) modified after46,47(edge length 100 m) and a process-based forest model (magenta-coloured line, mean, error bars, standard deviation). Figure 4: Model comparison for the estimated long-term impact of fragmentation on forests. Relative carbon loss per fragment over 30 years for different fragment sizes. Shown are results of a simple edge-effect model (turquoise) modified after [46] , [47] (edge length 100 m) and a process-based forest model (magenta-coloured line, mean, error bars, standard deviation). Full size image Figure 4 shows estimated relative carbon losses for different fragment sizes calculated with a simple forest-edge model and a process-based forest simulation model. The simple forest-edge model uses the remaining fraction of forest core area as the ratio of the forest-edge (100 m) area and the total forest area to estimate carbon losses (see Supplementary Methods ). Both models calculate the same trends ( Fig. 4 and Supplementary Fig. 3 ); the forest-edge model estimates higher carbon losses for smaller fragments. Results of the process-based forest model have been compared with forest inventories of fragments in the Brazilian Atlantic Forest [32] , [33] ( Supplementary Fig. 4 ). For all results presented, we use the loss curve based on the process-based forest simulation model ( Fig. 4 ). Biome-wide carbon loss We present the potential carbon losses due to the fragmentation added up for the Amazon Forest and the Brazilian Atlantic Forest—combining our long-term carbon loss estimates of single fragments with the fragment size distribution derived from remote sensing for the entire biomes ( Figs 1 , 2 , 3 , 4 , 5 ). Our analysis suggests that in addition to deforestation, the Brazilian Atlantic Forest may have lost approximately 69 Tg C (±14 Tg C) due to fragmentation effects only during 10 years of fragmentation ( Fig. 5 , area-based estimation). For the Amazon Forest, which is currently still far less fragmented than the Brazilian Atlantic Forest, the estimated overall carbon loss is 599 Tg C (±120 Tg C, MODIS data, area-based carbon loss estimate, Table 1 , Supplementary Table 1 ). If we take the explicit shape of fragments into consideration by including the ‘core area to total area ratio’ into the carbon loss estimate, the overall carbon loss increases to 775 Tg C (±155 Tg C, MODIS analysis, including shapes of fragments into the analysis, Table 1 , Supplementary Table 1 and Fig. 6 ). The spatial distribution of carbon loss due to fragmentation is highly heterogeneous within both biomes ( Figs 1 and 2 ). As the Brazilian Atlantic Forest is highly fragmented (see Table 1 and Supplementary Table 1 ), its biome-wide carbon losses yield an average loss of 0.43 Mg C ha −1 y −1 ( Table 1 ). Furthermore, we estimated that global carbon loss rate due to fragmentation in tropical forests worldwide ranges between 116 and 237 Tg C y −1 ( Supplementary Table 2 ). Sources of high uncertainties are the degree of fragmentation per biome or continent and the estimation of the amount of humid tropical forest area. 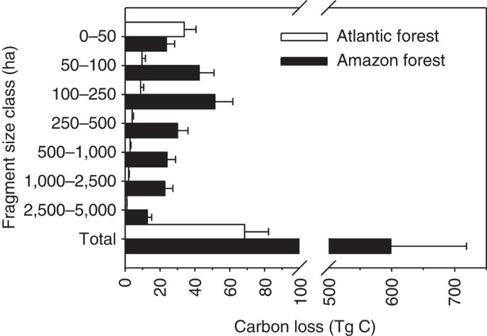Figure 5: Estimated average carbon loss in the Amazon and the Brazilian Atlantic Forests. Estimated average carbon loss in the Amazon Forest and the Brazilian Atlantic Forest over a period of 10 years. Results are shown for different fragment size classes (values for the total area of the corresponding size class; bar, C loss estimate per fragment size class; error bars, C loss uncertainty estimate of ±20%). Averages are calculated out of the 30 years simulation results. Figure 5: Estimated average carbon loss in the Amazon and the Brazilian Atlantic Forests. Estimated average carbon loss in the Amazon Forest and the Brazilian Atlantic Forest over a period of 10 years. Results are shown for different fragment size classes (values for the total area of the corresponding size class; bar, C loss estimate per fragment size class; error bars, C loss uncertainty estimate of ±20%). Averages are calculated out of the 30 years simulation results. 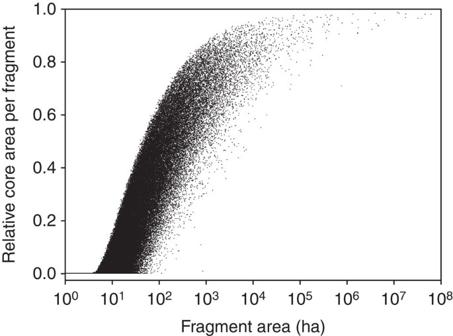Figure 6: Relative core area distribution of single forest fragments within the Amazon. Given is the ‘core area to total area ratio’ for each forest fragment of the Brazilian Amazon. Shown exemplary are data from 2009, PRODES dataset, for the Brazilian or Legal Amazon Forest respectively; analysis is based on 100 m edge width of the polygons. Full size image Figure 6: Relative core area distribution of single forest fragments within the Amazon. Given is the ‘core area to total area ratio’ for each forest fragment of the Brazilian Amazon. Shown exemplary are data from 2009, PRODES dataset, for the Brazilian or Legal Amazon Forest respectively; analysis is based on 100 m edge width of the polygons. Full size image On a global scale, the proportion of fragmented forest area is highly variable and not known in detail. Wade et al. [34] estimated that in Africa 18%, Asia 48%, Australia 30% and South America 14% of forests are affected by edge effects—they estimated edge area summing up all 1 km 2 pixels located in the edge area. Our own comparable MODIS analysis yielded 18.7% for the whole Amazon Forest, calculated as the percentage of edge area of total forest area at 1 km 2 resolution. Within the Brazilian Atlantic Forest, edge area adds up to 91% of the total forest area [35] using 1,000 m wide edges. Thus, we suggest that the Amazon Forest and the Brazilian Atlantic Forest can serve as exemplary cases of two extreme divergent degrees of tropical forest fragmentation, as fragmentation of the Brazilian Atlantic Forest and the Amazon Forest compare like positive and negative photographs: fragments in the Brazilian Atlantic forests are typically isolated islands, whereas fragments in the Amazon Forest typically include islands of deforestation—with the exception of the arc of deforestation in the southern and eastern Amazon. Concerning our estimation of the additional C loss due to fragmentation in the Amazon—599 Tg C (MODIS data, whole Amazon, area-based estimate), and 775 Tg C (for the shape-based estimate for the same data set), it reaches 7.5 to 40.0% of the estimated C emissions due to deforestation in the Amazon, when our results are scaled to the same time period (1 year) [10] , [14] , [15] , [26] (see Supplementary Table 3 ), or at least 54% of Brazil’s total emissions for energy and industry from 2005 ( Supplementary Table 3 ). Assuming that most tropical forests react similarly to fragmentation, and taking the Amazon Forest and the Brazilian Atlantic Forest as the upper and lower limits of possible degrees of habitat fragmentation at larger spatial scales, we estimated that additional annual fragmentation-induced carbon loss of 116 to 237 Tg C y −1 may result for all tropical forests [13] , [36] , [37] considered ( Supplementary Table 2 ). This amount corresponds to a ratio of 9% up to 24% of the estimated global annual C loss due to deforestation [11] , [13] , [15] , [38] . These additional C losses are due to the creation of edge areas, resulting from fragmentation processes, and are a relevant factor for the role of vegetation in the global carbon balance. The herein studied forest degradation process may increase the anthropogenic induced global annual C loss due to land use (until now, deforestation is the most important contributing process and accounts for approximately 10 to 15% of the total annual human C emissions [38] ). Several factors suggest that our estimates are conservative: first, edge effects may reach far more into forests than the 100-m wide edges our study used [32] , [33] , [35] , (for example, due to fire invading forests via edges [28] ); second, carbon loss in fragments with irregular shapes might be underestimated; third, comparing the analysis of MODIS and PRODES data for the Brazilian Amazon (see Supplementary Table 1 ) shows partly a scale issue, as PRODES captures small fragments of 1 ha, too. Thus, the results depend to some extent on the resolution. For example, we estimated for the Brazilian Amazon carbon loss being as high as 466 Tg C based on MODIS data (target resolution of around 250 m, see Methods), which increased to 514 Tg C based on PRODES data (based on Landsat data, see Methods and Supplementary Table 1 ); finally, our global C loss estimate does not yet include the shape-based C loss estimation; thus, our estimate is conservative with this respect. Since 1988, the forest area in the Amazon Forest affected by edge effects increased on average from 8.3 (ref. 39 ) to 18.7% (our MODIS analysis for the whole Amazon, data from 2009) on the basis of summing up 1 km 2 forest-edge pixels. This finding can be compared with other studies in the future at higher spatial resolution [40] . Despite globally increasing efforts to conserve tropical forests, fragmentation processes are likely to remain a highly relevant process affecting carbon dynamics in the Amazon Forest and other tropical forests. Our annual average of the fragmentation-induced additional C losses in the Brazilian Atlantic Forests during the first 30 years of fragmentation, 0.43 Mg C ha −1 y −1 , is comparable to other carbon losses or gains per hectare per year for other tropical forest studies: for tropical forests in Africa, Asia and America, average carbon gain was estimated to be 0.49 Mg C ha −1 y −1 between 1987 and 1997 based on 156 plot measurements [41] due to an increase of above-ground tree biomass. The 2005 Amazon drought led to C losses between 0.36 and 0.81 Mg C ha −1 y −1 at plot level [42] . Independent of the modelled scenario in detail, emissions would be much higher if the Amazon forests were fragmented to the same extent as the Brazilian Atlantic Forest [30] , [31] , [35] . In fact, this is a possible scenario [29] , [31] , given the ongoing deforestation in Brazil [40] . However, deforestation rates declined strongly in the last years, and this recent impact on additional C loss is still uncertain. Despite the fact that future patterns and intensities of land use remain unknown [14] , it seems highly probable that fragmentation processes will continue to play a relevant role in carbon dynamics in the Amazon Forest. As far as we know, this study provides the first estimate of biome-wide carbon loss due to forest fragmentation in two important Neotropical biomes, the Amazon Forest and the Brazilian Atlantic Forest, both biodiversity hotspots, by combining remote sensing, field data and process-based, dynamic, spatially differentiated modelling. We provide a generalizable strategy enabling the use of the outcome of local scale, dynamic ecological processes for larger scale spatial analysis. Our analysis shows that ecological changes at forest edges following fragmentation of tropical forests magnify carbon loss and contribute to the understanding of the role of vegetation within the global carbon cycle, even when making conservative assumptions for estimating carbon loss. Study design We combine biome-wide analysis of the distribution of tropical forest fragments via analysis of remote-sensing data for the Amazon and the Brazilian Atlantic Forest with carbon loss estimates of tropical forest fragments based on a simple edge-effect model and a process-based, dynamic forest model. Our satellite imagery analysis provided data on biome-wide spatial and size distributions of forest fragments, using Landsat data for the Brazilian Atlantic Forest [35] , MODIS and PRODES data for the Amazon Forest (details see below). We used these remote-sensing data to upscale model-based estimates of long-term carbon loss in fragments for the entire Brazilian Atlantic Forest and the Amazon Forest. A process-based, dynamic forest model [32] , [33] has been used to estimate long-term (any period as long or longer than 30 years) relative above-ground carbon losses for non-fragmented and fragmented forests. To translate relative losses in carbon estimates, we assume typical mean values for above-ground-stored carbon in trees in undisturbed forests (125 Mg C ha −1 for the Brazilian Atlantic Forest [32] , [33] and 170 Mg C ha −1 for the Amazon [13] , for more details see below). Analysis of forest fragment distribution Forest fragment distribution within the Brazilian Atlantic Forest was analysed based on a Brazilian Atlantic Forest vegetation map from the year 2005 ( www.sosma.org.br and www.inpe.br ) produced by SOS Mata Atlântica/INPE (2008) (ref. 35 ). The map was constructed by analysis of TM/Landsat-5 (TM) and CCD/CBERS-2 (CCD), which was first classified into vector format, and then converted to raster, with a 50-m spatial resolution. In contrast to the Brazilian Atlantic Forest, fragments in the Amazon Forest were mapped by using the MODIS satellite data classifying a 16-day Enhanced Vegetation Index (MODIS-EVI with an initial spatial resolution of 250 m). In addition, the tiled PRODES data set [43] , [44] , [45] (based on Landsat data), whose spatial dimensions correspond to the Brazilian or Legal Amazon, respectively, was also used. Due to the presence of clouds, two different maps were generated—the first, considering clouds as non-forest and the second, considering them as forest ( Supplementary Table 1 ). Simulation model From these maps, we used the variables ‘number of patches per fragment size class’, ‘total area of fragmented forest per size class’ and the ‘core area to total area ratio of each fragment’ (relative core area) to upscale patch-level estimates of carbon loss. Carbon losses in the border area of forest fragments are estimated with two methods: first, with a simple edge-effect model, which is based on estimating the relative core area of a forest fragment. The relative core area itself depends on the size of the border area and the fragment shape [46] , [47] ( Supplementary Methods ). Second, we obtained carbon loss in the border area of forest fragments with the dynamic, process-based forest-growth model FORMIND [32] , [33] and compared results for single forest fragments with the results of the simple edge-effect model. FORMIND models tree growth, seed dispersal, recruitment, mortality, competition for light and space and disturbances by grouping trees into functional types [32] , [33] . FORMIND is an individual- and process-based forest model, which has already been applied and tested in many different regions of the tropics [32] , [33] ( Supplementary Methods ), capturing not only the main ecological processes, but also the spatial differentiated degradation of forest (for example, due to fragmentation), and the subsequent regrowth on that patch, too. We parameterized the model such that it yielded on average an above-ground-stored carbon in live trees of 125 Mg C ha −1 , as estimated empirically for non-fragmented forests of the Brazilian Atlantic Forest [32] , [33] , [48] , [49] , and for the Amazon Forest we applied 170 Mg C ha −1 for undisturbed forests [13] . Implementation of forest-edge effects [32] , [33] , especially increased mortality at forest edges, was inspired by the results of the Amazon fragmentation project [21] , [22] , [28] , [29] , [31] . Carbon loss estimation We simulated forest patches for sizes between 1 and 2,601 ha for 200 years and used the annual and the accumulated biomass and carbon loss over 30 years as main response variables. Then, we derived a statistical relationship of the simulated relative above-ground carbon loss in trees within 30 years against fragment size by a non-linear regression to extrapolate our simulation results to fragment sizes that have not been simulated. Using results of the forest model and the described regression analysis, we estimated carbon loss for each fragment identified by satellite imagery analysis from the Amazon Forest (for both MODIS and PRODES datasets) and the Brazilian Atlantic Forest. The PRODES dataset is based on Landsat data. For the Amazon data, we included the shapes of the real fragments into our analysis via using their ‘core area to total area ratio’ and equating this ratio with that of the simulations. We obtained the biome-wide ‘total carbon loss over 30 years’ estimates by integrating the total losses of all fragments. To relate carbon loss caused by fragmentation to the estimated annual carbon losses caused globally and within the Amazon by land use change, we calculated the 10 years and yearly average, and the average C loss in Mg ha −1 y −1 for all fragments per biome as one basis for the global estimate. Remote sensing of the Amazon Basin The study area included all Brazilian states covered by Amazonian Forests (Amazonia Legal) as well as the Amazon Forest located in neighbouring countries. The total size of the study area was 9.4 million km 2 . Forest fragments of the complete Amazon Basin were mapped in 2009 using the 16-day MODIS Enhanced Vegetation Index (EVI, sinusoidal projection) with a resolution of 250 m for 20 different dates spanning the period Jan. 17th to Nov. 17th 2009 to obtain seamless and cloud-free coverage. These data were projected with a target resolution of around 250 m to the South American Albers Equal Area Projection ( http://spatialreference.org/ref/esri/102033/ ), which is well-adapted for area analysis. To reduce noise, the minimum mapping unit was set to 3 × 3 pixels or 36 ha. The focus observation period was in October and November 2009; data collected between January and August 2009 were only used if there were no data available for the focus time period due to cloud cover. Threshold values to distinguish forest cover from non-forest were determined using MERIS GlobCover 2.2 for 2005 (ref. 50 ) and the Brazilian PRODES dataset [43] for yearly deforestation ( www.inpe.br ). All analyses were performed in Albers Equal Area projection for South America, and all MODIS landscape analysis has been performed with GRASS [51] . PRODES [43] , [44] , [45] data of 2009 have been also analysed, and were acquired from the PRODES INPE website ( http://www.obt.inpe.br/prodes/index.php ). Maps were originally in vector format, but the files were first merged into a unique file, and then converted to raster format. From this unified raster data, two vegetation maps were generated, one considering clouds as forest, and another one considering them as non-forest ( Supplementary Table 1 ). The coordinate reference system used was the Albers Equal Area. All landscape statistics were then calculated using ESRI ARCGIS ( www.esri.com ) with the Patch Analyst Extension ( http://www.cnfer.on.ca/SEP/patchanalyst/ ), except for the calculation of core areas, which was done in the Quantum GIS environment ( http://www.qgis.org/ ). The forest fragment classification of PRODES data has been compared against the MODIS classification ( Supplementary Table 4 ). Accuracy assessment of the Amazon map The regional classification of Globcover 2.2 was used for accuracy assessment of forest fragments. As Globcover for 2009 was not yet available, the Globcover for 2005 was used which was regarded as the highest quality and highest resolution land cover product available for Amazonia [50] . From this reference map, the categories 40: ‘Closed to open (>15%) broadleaved evergreen or semi-deciduous forest (>5 m)’, 41: ‘Closed (>40%) broadleaved evergreen and/or semi-deciduous forest (>5 m)’, and 160: ‘Closed to open (>15%) broadleaved forest regularly flooded (semi-permanently or temporarily)—Fresh or brackish water’ were used as equivalent to forest cover to calculate Kappa [52] and G (per cent correctly classified pixels) statistics for the detection of forest fragments. The Kappa value for forest fragments was 0.677 and for non-forest areas it was 0.748, yielding an overall Kappa value of 0.711. Overall, 87.3% of all pixels were correctly classified. Amazon Forest fragmentation landscape metrics Two different parameters of forest fragments were estimated and analysed: fragment size, and edge area ( Supplementary Table 5 ). With fragment size we determined the amount of fragmented forest area and the number of fragments for different size classes. 68.4% of the study area, consisting of 77,038 fragments, was covered by forest. The two largest fragments covered 93.6% of the forested area. 53.8% of all fragments where smaller than 100 ha. Edge area was calculated as the amount of forest area exposed to edge effects for different edge widths. 4.98% of the forest area was less than 250 m away from any nearest edge, 18.7% of the forest area was less than one km away from the nearest edge. The largest distance to the nearest edge was 98.5 km. Remote sensing of the Brazilian Atlantic Forest Forest cover and the spatial distribution of fragments of almost the entire original extent (94%, 1,395,849 km 2 ) of the Brazilian Atlantic Forest were analysed by Ribeiro et al. [35] based on a Brazilian Atlantic Forest vegetation map from the year 2005 produced by SOS Mata Atlântica/INPE (2008, www.sosma.org.br and www.inpe.br ). The map was projected to the Albers projection and the South America 1969 Datum and was constructed by visual interpretation of TM/Landsat-5 (TM) and CCD/CBERS-2 (CCD), viewed as colour compositions on a digital orbital image mosaic with bands TM3 (red region in the blue filter), TM4 (near infrared, NIR, in the red filter) and TM5 (short wavelength infrared, SWIR, in the green filter) for Landsat-5, CCD-2 (green in blue filter), CCD-3 (red in green filter) and CCD-4 (NIR in red filter) for CBERS-2. This map was in vector format and included three main vegetation classes, grouping several physiognomically and floristically distinct forests: first, forests (including coastal forests, Araucaria mixed forests and semi-deciduous forests), second, ‘Restinga’ forests (lowland forests on sandy soils near the coast) and third, mangrove forests. Only the first vegetation type was analysed for extracting the fragmentation patterns. The mapping scale was 1:50,000, which was converted to raster, with a 50-m spatial resolution, to improve metric computation. The ‘forest’ class includes secondary forests at intermediate to advanced successional stages, but not early successional stages. A complete description is given in Ribeiro et al. [35] Carbon loss maps We analysed the overall biomass and carbon loss and its spatial distribution for the 245,173 forest fragments of the Brazilian Atlantic Forest and the 77,038 fragments of the Amazon Forest (MODIS), and the 389,140±78,787 fragments of the Brazilian Amazon (mean based on both maps of the PRODES dataset, Supplementary Table 1 ) employing a logistic regression to interpolate the forest simulation data to the size of each of the identified fragments (equation 1): where a and b are dimension-less parameters, the parameter c is in (ha), y 0 (%) is the relative minimum biomass, x (ha) is the area of habitat patches and B (%) the relative above-ground biomass in the forest fragment compared with the undisturbed forest. The estimated values for the parameters were: y 0 =34.9447, a =63.5742, b =0.687, c =10.459 ha (non-linear regression Sigmoidal Hill, R 2 =0.99). All carbon values were then obtained by scaling them with the estimates of above-ground-stored carbon for the correspondent region (125 and 170 Mg C ha −1 , respectively, assuming C content being 50% of biomass). We based our calculations on published values for above-ground-stored carbon in trees for the Brazilian Atlantic Forest [32] , [33] , [48] , [49] (using the estimates for above-ground-stored carbon in live trees of approximately 125 Mg C ha −1 for the Atlantic Forest and 170 Mg C ha −1 for the Amazon [13] ). We used these values as exemplary to analyse biome-wide consequences of fragmentation on carbon loss and are aware about the heterogeneities and uncertainties concerning the spatial distribution of stored carbon in Neotropical forests [7] , [15] , [53] . However, we decided to use biome-wide average estimates as long as current maps of local carbon densities show substantial differences among each other [54] , [55] . Therefore, we assumed an envelope of uncertainty for our C loss estimates of ±20%. Then we calculated for the simulated forest fragments the ‘core area to total area ratio’ ca sim , which is affected by the size of the total edge area of each fragment. The biomass and carbon deficit of each forest fragment was then estimated by using the result of that simulated forest fragment, which has the same ‘core area to total area ratio’ of the monitored fragment ca emp . For the calculation of the ‘core area to total area ratio’ ca sim , we used the following equation 2: where el is the edge length of the simulated forest fragment expressed in units of 100 m defining the edge area and ca emp is the ‘core area to total area ratio’ of the real forest fragment. By using this edge length, we calculated the area of the simulated fragment with the same ‘core area to total area ratio’ (relative core area) ca sim as the real forest fragment ( ca emp ) for estimating C loss for each real fragment considering its shape. Then we estimated, for each forest fragment, the biomass and carbon loss (in Mg ha −1 ) by subtracting the estimated biomass from the upper limit (above-ground biomass per ha for large undisturbed forest fragments), and summed up the values for each fragment size class (in Tg C). For the estimation of the carbon loss per fragment based on its shape, equations (1) and (2) were used, for the carbon loss estimate based on area, only equation (1) was used. For illustrating the results in Fig. 3 and Fig. 5 , all forest fragments were classified into fragment size classes (ha). As additional parameters, we analysed the ‘ratio between area size and squared perimeter’ and the ‘Didham shape index’ [47] an extension of the shape index developed by Laurance and Yensen [46] . Biome-wide estimation of carbon loss We performed a non-linear regression using a logistic function of above-ground tree biomass and carbon loss as a function of fragment size (assuming carbon content to be 50% of biomass). Forest biomass obtained in the simulations was compared with empirical biomass estimates for fragments and forests of the Plateau of São Paulo [32] , [33] , [49] . Biome-wide estimation of long-term carbon loss was calculated by combining the results of the simulation experiments with the biome-wide forest fragment distributions obtained via satellite image analysis of a resolution of 50 m for the Brazilian Atlantic Forest [35] and 250 m for the Amazon Basin (MODIS data, own analysis, see above for method) and based on Landsat data for the Brazilian Amazon (PRODES [43] , [44] , [45] data, own analysis) using the ‘number of fragments per fragment size class’, ‘total area cover per fragment size’, and ‘the core area to total area ratio’. To present the calculated maps of biomass loss, we use the ‘isolated fragment’ scenario (see Supplementary Methods ) after 30 years of fragmentation. The estimation of carbon loss due to fragmentation assumes that every fragment has been fragmented at the same time at the beginning of each simulation, to be able to analyse the edge effects of fragmentation for a whole biome, as at present, robust models, which estimate either the present fragment age, the history of a fragment or its prospective age, are lacking. We further assumed that the neighbourhood of the fragment did not change during the simulation, as it is not yet possible to dynamically track the complete land use change of a biome. The analysis is then presented with the 10 years and 1 year average for the whole biome and the average C loss per hectare per year. Please be aware that these averages are scenario specific and should not be taken as short-term rates. Annual global carbon loss estimation for tropical forests For a first estimation of annual global carbon loss from humid tropical forests after Laurance et al. [56] we refer to the figures of Wade et al. [34] , as other data are lacking (equation (3)). The continental estimates provided by Wade et al. [34] were summed up, providing an estimated average degree of global forest fragmentation of 28%. We normalized our result—the average carbon loss per hectare per year for the first 30 years for the Brazilian Atlantic Forest ( Table 1 , average degree of fragmentation: 91%) to the relative C loss compared with the carbon content of the reference forest (125 Mg C ha −1 ) and to 1% degree of fragmentation. Then, we estimated the additional C loss per continent proportionally to the degree of fragmentation of each continent provided by Wade et al. [34] , the reference biomass for above-ground-stored C in trees in undisturbed forests [13] , and the total area for humid tropical forests (if available) for the given continent/biome [13] , [36] , [37] , [57] . In addition, we assumed an envelope of uncertainty of ±5% to the fragmentation degree at continental level (see Supplementary Table 2 ). with Cl c being the C loss estimate per continent/biome, C lossAFn being the normalized mean C loss after 30 years of fragmentation in the Brazilian Atlantic Forest for 1% degree of fragmentation; df c is the corresponding degree of fragmentation of the estimated biome/continent, A TFc is the continental humid tropical forest area ( Supplementary Table 2 ) and C abc is the reference biomass per continent [13] . How to cite this article : Pütz, S. et al. Long-term carbon loss in fragmented Neotropical forests. Nat. Commun. 5:5037 doi: 10.1038/ncomms6037 (2014).